Shared developmental programme strongly constrains beak shape diversity in songbirds The striking diversity of bird beak shapes is an outcome of natural selection, yet the relative importance of the limitations imposed by the process of beak development on generating such variation is unclear. Untangling these factors requires mapping developmental mechanisms over a phylogeny far exceeding model systems studied thus far. We address this issue with a comparative morphometric analysis of beak shape in a diverse group of songbirds. Here we show that the dynamics of the proliferative growth zone must follow restrictive rules to explain the observed variation, with beak diversity constrained to a three parameter family of shapes, parameterized by length, depth and the degree of shear. We experimentally verify these predictions by analysing cell proliferation in the developing embryonic beaks of the zebra finch. Our findings indicate that beak shape variability in many songbirds is strongly constrained by shared properties of the developmental programme controlling the growth zone. Bird beaks are three-dimensional structures that show a tremendous diversity in shape and size. They profoundly affect survival and play a major role in the avian radiation as the most diverse group of land vertebrates [1] . Their adaptive significance makes them a very useful developmental model for understanding mechanisms of morphological diversification and principles of evolution of biological shapes [2] . Over a century of ecological research on birds showed that differing beak shapes help to adapt to different food sources, and it is often argued that beak shape is optimized for specialized foraging [3] , [4] . Interestingly, an alternative point of view [5] suggests that beak shape diversity mainly results from morphogenetic processes independent of adaptation, with constraints being largely imposed by the beak developmental programme. Within this hypothesis, beak phenotypic variation and morphological adaptation would be limited or strongly biased by the structure and dynamics of its developmental programme [6] . Both extrinsic and intrinsic factors are expected to play a role in shaping morphological diversity. However, untangling their relative importance is difficult, since details of the beak developmental programme are only known in a small number of species. In this study, we investigate how strongly diversity is constrained by the programme of beak development shared across birds. To quantify morphologies and the associated diversity, we investigate what transformations are necessary to map the beak shapes of different birds onto each other, an approach first introduced by D'Arcy Thompson [7] . We focus on songbirds (Suborder Passeri, Order Passeriformes), because they are the largest group of birds, composed of over 4,000 species, and exhibit extraordinary diversity of feeding habits and corresponding beak morphologies [1] . They are an excellent model for evaluating the role of possible developmental constraints in the evolution of avian beak morphology. The recent discovery that the developmental mechanism underlying beak shape diversity within Darwin’s ground finches ( Geospiza, Thraupidae) results from the combined action of several morphogens that independently control the depth/width and length of the prenasal cartilage ( pnc ) and the premaxillary bone ( pmx ) [8] , [9] , [10] , [11] , [12] suggested that their beak shapes might superimpose onto a single common shape after normalizing each axis with its corresponding scale. We recently demonstrated that this is in fact the case, and moreover that the beaks of species in genera closely related to Geospiza , like the vegetarian, tree, Cocos or warbler finches, do not collapse onto the Geospiza beak shape under scaling, indicating that their beak shape is fundamentally different from the Geospiza shape [13] . However, by extending the class of transformations to include shear along the length component of the beak, the beak shapes across all these genera collapse onto the Geospiza shape [13] . That is, under a subset of affine transformations, all these beak shapes can be mapped onto each other. Here we examine the relevance of this observation in songbird beaks more generally by analysing the beak profiles obtained from lateral pictures of museum specimens of 173 different songbird species. We broadly sampled representatives of the tanagers (Thraupidae), the cardinals (Cardinalidae) and the weaver finches (Estrildidae). The tanager family in particular is one of the largest and most diverse families of songbirds in terms of beak shapes and feeding habits (this group includes Darwin’s finches [14] ), while the estrildid finches include the zebra finch ( Taeniopygia guttata ), the most common model songbird species used for morphological, behavioural and genetic studies. In combination, the species we study here cover most of the range of beak shapes and diets found in all songbirds. We show that all of these beak shapes are equivalent under affine transformation, with the midsagittal cuts of the beaks well fit by a three parameter family of conic sections, a strikingly simple set of geometric shapes. To probe why the observed beak shape variation is characterized by such a small set of shapes, we carry out a mathematical analysis of possible developmental programmes that can produce beaks shaped as conic sections: the solution places strong limitations on these programmes. We find that the size and time dependence of the growth proliferation zone that gives rise to the beak shape must obey strict power laws. We then test and verify these predictions in zebra finch T. guttata embryos by studying dynamics of cell proliferation using 5-ethynyl-2′-deoxyuridine (EdU) labelling on medial sections of the upper beak during several key developmental stages when the beak forms and undergoes morphogenesis. Taken together, the results suggest that morphological diversity seen in songbird beaks largely arises from and is probably limited by the particular features in the existing developmental programme. Quantifying beak shape diversity The avian bill comprises the upper and lower beaks, which develop largely independently [8] , and many studies, including this one, focus on the morphologically more diverse and developmentally better understood upper beak. This structure is the critical structural and biomechanics component for mastication and other bird bill functions that experiences strong levels of selective pressure [3] , [15] . Some of the most important beak shape parameters, such as depth, length and curvature can be readily studied on two-dimensional profile images. These considerations led us to consider only the top profile of the upper beak for three individuals from each species; this is not restrictive as the upper beak shape reflects the functional biomechanical properties of the entire bill [3] and upper beak shape diversity is highly predictive of the shape of the entire midsagittal section. Our previous study [13] demonstrated that within the genus Geospiza , where computed tomography scans were available, the scalings predicted by the shape of the upper contour of the upper beak also apply to the shape of the entire midsaggital section of the upper beak. To determine whether two given (upper) beak shapes y 1 ( x ) and y 2 ( x ) represent the same shape under a given transformation, we let denote the transformed shape, rescaled by s l along the length and by s H along the height dimension and compute two metrics quantifying the difference in their shape and their derivative profile [13] . If there is a global minimum in E s and E d for a given set of s l and s H , then the values of E s and E d (their residuals) measure how closely the two shapes y 1 ( x ) and y 2 ( x ) are related by scaling transformations. We perform a pairwise comparison of the upper beak shapes of 173 bird species spanning a significant section of Passeroidea ( Fig. 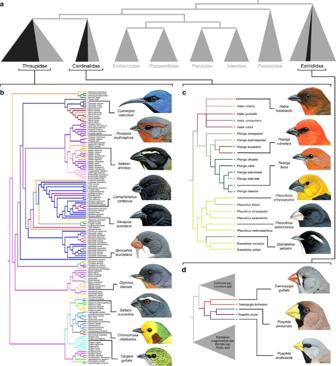Figure 1: The phylogenetic and morphometric structure of beak shapes. (a) Major families in Passeroidea, sized according to number of species in the family (grey triangles). Proportion of species sampled in our shape analysis are represented in black. (b–d) Maximum likelihood phylogeny of Thraupidae/Cardinalidae /Estrildidae, respectively, indicating diversification of beak shape across the phylogenetic history of the group, with illustrations of beak shape for representative species to show range of morphological diversity. Colours represent group shapes of beaks mapped onto the phylogeny using maximum likelihood. Species in the same colour collapse onto each other with scaling alone, all shapes collapse under shear. Bird images reproduced with permission from ref.50. 1 , Supplementary Table 1 ). 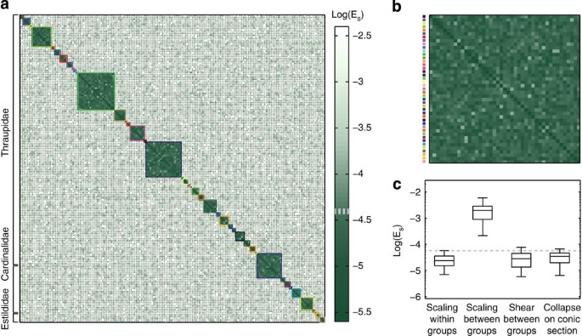Figure 2: The hierarchical collapse of beak shapes onto each other under scaling and shear. (a) Heat map ofEsresulting from pairwise comparisons of all beak shapes in the phylogeny, scaling one beak shape onto another. Crosses (X) indicate pairs of species whose beaks do not collapse via scaling transformations, as there was no minimum inEsas a function of the scaling factors. Note the large blocks where the residual is small—these are the scaling groups. (b) Residuals for the collapse of the different scaling groups found inawhen rescaled using shear transformations. The colours of the rows correspond to the block colours ina. Note the magnitude of the residuals on shear collapse are similar to those for the scaling groups. (c) Box plots (median, first and third quartile and 2nd and 98th percentile) showing quality of collapse (in terms ofEs) for the different levels of similarity presented in panelsaandb. Note that the quality of scaling within groups, shear between groups and collapse of all beak shapes on conic sections is on the same order of magnitude as our precision of measurement for beak shapes (set by the resolution of modern digital cameras, represented by a grey dashed line). Figure 2a shows a heat map of the residuals for these pairwise comparisons, with the different species clustered according to their similarity in beak shape. The heat map clearly identifies 43 morphological groups, represented by colours, within which the beak shapes differ only by their scales. Scaling transformations thus account for a substantial part of the variation observed in songbird beak shapes by reducing the complexity from 173 original beak shapes to 43 different (group) shapes. The character mapping analysis onto the molecular phylogeny also detects 12 cases of convergence of the group shapes in the Thraupidae alone ( Fig. 1 , Supplementary Fig. 1 ). If we extend the space of transformations to include shear along the length dimension, then we observe that all the beaks’ shapes collapse, as shown in the heat map in Fig. 2b . The beak shapes can be mapped exactly (within the precision provided by modern digital cameras) onto each other under scaling and shear, characterized by precisely three parameters: the height and length ( s l and s H , respectively) for the scaling transformation and an additional parameter τ measuring the degree of shear. This pattern of hierarchical collapse of shapes is represented in Fig. 3 . Figure 1: The phylogenetic and morphometric structure of beak shapes. ( a ) Major families in Passeroidea, sized according to number of species in the family (grey triangles). Proportion of species sampled in our shape analysis are represented in black. ( b – d ) Maximum likelihood phylogeny of Thraupidae/Cardinalidae /Estrildidae, respectively, indicating diversification of beak shape across the phylogenetic history of the group, with illustrations of beak shape for representative species to show range of morphological diversity. Colours represent group shapes of beaks mapped onto the phylogeny using maximum likelihood. Species in the same colour collapse onto each other with scaling alone, all shapes collapse under shear. Bird images reproduced with permission from ref. 50 . Full size image Figure 2: The hierarchical collapse of beak shapes onto each other under scaling and shear. ( a ) Heat map of E s resulting from pairwise comparisons of all beak shapes in the phylogeny, scaling one beak shape onto another. Crosses (X) indicate pairs of species whose beaks do not collapse via scaling transformations, as there was no minimum in E s as a function of the scaling factors. Note the large blocks where the residual is small—these are the scaling groups. ( b ) Residuals for the collapse of the different scaling groups found in a when rescaled using shear transformations. The colours of the rows correspond to the block colours in a . Note the magnitude of the residuals on shear collapse are similar to those for the scaling groups. ( c ) Box plots (median, first and third quartile and 2nd and 98th percentile) showing quality of collapse (in terms of E s ) for the different levels of similarity presented in panels a and b . Note that the quality of scaling within groups, shear between groups and collapse of all beak shapes on conic sections is on the same order of magnitude as our precision of measurement for beak shapes (set by the resolution of modern digital cameras, represented by a grey dashed line). 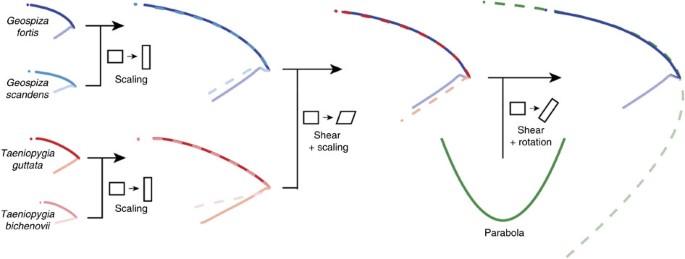Figure 3: The basic pattern of beak shape diversity. On small phylogenetic scales, beak shapes collapse under scaling alone (for example, the twoGeospizaspecies on the top left), creating groups of similar beak shapes (represented by colours). These group shapes in turn collapse onto each other under shear in their length direction. Specifically, all group shapes collapse onto the shape of the blue coloured group. This blue coloured group can be approximated to an extremely high precision as a section of a parabola, as shown on the right. The combination of this hierarchical collapse under scaling and shear onto the blue coloured group, and the collapse of the blue coloured group on a parabola lead to the conclusion that all beak shapes considered here are conic sections. Full size image Figure 3: The basic pattern of beak shape diversity. On small phylogenetic scales, beak shapes collapse under scaling alone (for example, the two Geospiza species on the top left), creating groups of similar beak shapes (represented by colours). These group shapes in turn collapse onto each other under shear in their length direction. Specifically, all group shapes collapse onto the shape of the blue coloured group. This blue coloured group can be approximated to an extremely high precision as a section of a parabola, as shown on the right. The combination of this hierarchical collapse under scaling and shear onto the blue coloured group, and the collapse of the blue coloured group on a parabola lead to the conclusion that all beak shapes considered here are conic sections. Full size image To further quantify the diversity of shapes, we fit polynomial functions to the beak profiles and search for the beak shape with the simplest functional form (see Supplementary Fig. 2 ). This turns out to be Geospiza in the Darwin’s finches, which are fit well to within the error of our methods for recording shapes by a parabola y = ax 2 + bx . The shear collapse of all other songbird beaks onto this shape implies that all beak profiles are well fit by this equation after sending x → s l x + τy and y → s H y . Thus, all beak shapes are well fit by an equation of the form The midsagittal sections of songbird beaks investigated here are all conic sections. Features of developmental programmes are strongly constrained All beak shapes are the direct product of a developmental process during which mesenchyne derived from neural crest cells undergoes differentiation to produce facial skeleton. The upper beak and face are formed by five different primordia: the central frontal nasal mass, the paired lateral nasal and maxillary prominences [8] . All available evidence argues that the midsagittal section that we study in this report is derived from the frontal nasal mass [16] , [17] , [18] , [19] . One of the best-understood model systems of beak evolution in songbirds is Darwin’s finches [11] , [12] , [20] . In this group, the two most important skeletal structures whose combined morphogenesis defines the shape of the adult beak are the pnc during early and mid-stages of embryonic development followed later in development by the medial pmx , which represent independent developmental modules controlled by different morphogens, and which play distinct roles in shaping beaks of different species [14] , [20] . For example, previous studies on beak development in Geospiza (Darwin’s finches) revealed that signalling molecules, such as Bmp4 and Calmodulin, control the depth/width and length of the pnc , respectively, while TGFβIIr, β-catenin and Dkk3 together control the depth and length of the pmx [11] , [12] , [13] , [14] , [20] . The size and shape of the growing beak is determined largely by the inherent ability of the neural crest cells to receive and interpret local signalling information, as was demonstrated by the cranial neural crest transplantation experiments in quails and ducks [9] . If neural crest cells in a duck embryo are replaced by those from the quail embryo, the resulting beak looks quail like, reflecting the origin of the neural crest cells and vice versa . Certain parameters of beak morphology, for example its depth, can be affected by different tissue modules and regulatory molecules in different species [20] . In all bird species examined, the expression patterns of regulatory molecules controlling beak mophogenesis are most prominent around a small focal region, close to the rostral tip of the growing beak [21] , and earlier studies of beak growth in chicken and duck embryos show that this area is also the main region of cell proliferation in the upper beak primordium [10] . This mode of growth can be modelled by considering a relatively simple scenario: the induction by morphogens generates a group of dividing cells localized near the rostral tip of the growing beak, the highly defined growth zone. This group of cells changes its shape, size and position as the beak grows. We can describe the shape of the growth zone by the solution to G ( η , ξ ) where and . Here ( x 0 , y 0 ) are the locations of the centre of the growth zone and l ( t ) is the size of the zone. With this definition, the final shape of the beak is essentially given by the envelope of the growth zone over time, if cell rearrangement during growth is not significant. The envelope for these growth zone shapes is given by ∂ t G =0. Using this framework, we can ask what the observed invariances from our analysis of beak shapes imply about the growth process. Under what conditions do these laws have solutions that can only be equation (1)? To understand this, we note that the most prominent feature of bird beaks is their sharp tip, which requires the size of the growth zone l ( t ) to shrink to size zero in finite time. We can only produce shapes that are conic sections by choosing the growth zones to be homogenous functions of time, namely, x 0 ( t )= α ( t *− t ) q , y 0 ( t )= β ( t *− t ) q and l ( t )=γ(t*−t) p , where t * is the time when beak growth ends. Different scaling groups of beak shapes can then naturally be generated by modifying the prefactors α , β and γ for the same exponents p and q (see Supplementary Fig. 3 ). Given these laws for the size and movement of the growth zone, the envelope for any polynomial function in η and ξ will simultaneously obey G ( η , ξ ) and ∂ t G =0, or where and . If G is a polynomial of degree n , then equation (2) is a polynomial of degree n −1. Bezout’s theorem then implies that the system has at most n ( n −1) solutions of the form where Γ, Θ are constants, if α , β , γ , p , q are chosen. We can express these solutions in terms of the original variables as for example, Subtracting these, and using the power law forms for x 0 ( t ), y 0 ( t ) and l ( t ) then implies with A , B = f ( p , q , α , β , γ ) depending on the form of G . This demonstrates that the envelopes of growth zones are exactly conic sections in agreement with equation (1) only for scaling exponents p / q =2. Only a very small class of developmental laws for the growth zone allows the resulting beak shapes to be exclusively conical sections, as demanded by our empirical observations. These dynamics must be satisfied individually for both the upper and lower profile of a midsagittal beak section. Even for a single profile, the invariance of beak shapes sets the exponents of the power laws ( p and q ) and the precise shape of the profile forces values for all other parameters ( α , β and γ ). Since the required values for these parameters will generally be slightly different for the upper and lower profile, both can only be satisfied simultaneously if we allow for an additional degree of freedom in allowing the shape of the growth zone to be anisotropic. We have investigated this with Monte–Carlo calculations, which show that there is still some freedom in the set of growth zone shapes that can generate a given combination of upper and lower profile (see Supplementary Fig. 3 ) while still preserving p / q =2. Under the assumption that the growth zone shape G ( η , ξ )=0 is preserved in time, we find a one-parameter family of growth zone shapes that are consistent with a given upper and lower beak profile. Thus, the observation that beak profiles of songbirds are conic sections not only precisely fixes the dynamics of growth zone development but also constrains its potential shape at each embryonic phase. Experimental verification On the basis of the theoretical results derived above, any universal law for the growth zone dynamics satisfying p / q =2 could generate the patterns of beak shape diversity observed in nature. The simplest scenario has p =1, which corresponds to the location of the centre of the growth zone moving with constant velocity. This would occur if the division rate of cells within the growth zone is constant in time, and the centre of the growth zone is pushed forward by the dividing cells. With p =1, we must have q =1/2, which implies that the largest dimension of the growth zone decreases to zero as t 1/2 . We test these predictions by measuring the size and position of the growth zone in embryos of zebra finch ( T. guttata) undergoing morphogenesis, since their adult beak shape collapses under scaling and shear onto the Geospiza shape and all other studied songbirds (see Fig. 3 ). We analyse midsagittal sections of the upper beak from stage E5 (embryonic day 5), when the growth zone can first be clearly delineated at the rostral tip of the developing beak, to E9, when the growth zone is no longer visible. All sections are stained to show dividing cells (with injection of EdU cell proliferation marker, shown in green) as well as cell nuclei (blue) and either cartilage precursor (with Lectin Peanut agglutinin (PNA), shown in magenta) or established cartilage (with Col2, shown in magenta). The growth zone is clearly identifiable as a concentrated region of dividing cells close to the tip of the developing beak (see Fig. 4a ). We use a simple filter and thresholding method to determine the size of the growth zone at these different developmental stages (see Supplementary Fig. 4 for details). 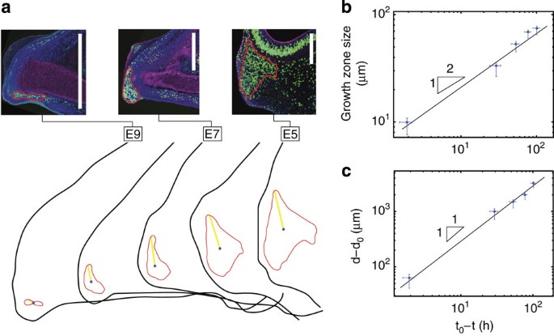Figure 4: Experiment testing the time development of the growth zone in developing zebra finch embryo beaks. (a) Snapshots of growing beak for stages E5–E9, showing its outline (black), the size of the growth zone (red), its centroid (blue) and the relevant length scale for shaping the upper beak profile (yellow). All measures of the growth zone are derived from midsagittal cross-sections of zebra finch embryo beaks, stained to show cell nuclei (in blue) and dividing cells (in green). Areas with a high density of dividing cells are defined as the growth zone (red outline). Scale bar, 500 μm. (b) The dimension of the growth shrinks as (t*−t)1/2, consistent with theoretical predictions. (c) The distanced−d0of the centre of the growth zone from the point where upper and lower beak meet increases as (t*−t), consistent with theoretical prediction. Error bars along the abscissa represent uncertainty in timing within the stages E5–E9 and errors along the ordinate represent variation with respect to the threshold used to separate EdU staining from the background. Figure 4b shows that the largest dimension scales with the expected t 1/2 dependence in time ( q =0.52±0.05), as predicted by the theoretical framework. Figure 4: Experiment testing the time development of the growth zone in developing zebra finch embryo beaks. ( a ) Snapshots of growing beak for stages E5–E9, showing its outline (black), the size of the growth zone (red), its centroid (blue) and the relevant length scale for shaping the upper beak profile (yellow). All measures of the growth zone are derived from midsagittal cross-sections of zebra finch embryo beaks, stained to show cell nuclei (in blue) and dividing cells (in green). Areas with a high density of dividing cells are defined as the growth zone (red outline). Scale bar, 500 μm. ( b ) The dimension of the growth shrinks as ( t *− t ) 1/2 , consistent with theoretical predictions. ( c ) The distance d − d 0 of the centre of the growth zone from the point where upper and lower beak meet increases as ( t *− t ), consistent with theoretical prediction. Error bars along the abscissa represent uncertainty in timing within the stages E5–E9 and errors along the ordinate represent variation with respect to the threshold used to separate EdU staining from the background. Full size image Comparisons between different tissue sections at the same developmental stage and the same (midsagittal) plane indicate that the distance of the growth zone to the region where upper and lower beak meet is very uniform. This distance is, therefore, a good measure for determining the speed with which the growth zone advances relative to a fixed point outside the developmental module. For each growth zone as determined above, we find its centroid, and measure the distance from the meeting point between upper and lower beak and this centroid. Figure 4c shows the results of this analysis, which demonstrate that the speed of advance for the growth zone is indeed linear ( P =0.98±0.08), and thus based on these experimental results, which agrees well with the theoretically predicted value of The work described herein demonstrates that the shapes of songbird beaks’ profiles are a subset of conic sections. This is only a small region of the possible morphological parameter space that the shapes of bird beaks could occupy, thus supporting the hypothesis that the beak shape of songbirds is strongly constrained by its developmental programme. We demonstrated a strong correlation between the shape of a developing beak and the dynamics of the growth zone that shapes it. This, in turn, suggests that there are additional strong constraints on growth zone dynamics by regulatory processes that can be investigated more directly in future experiments. Our growth model only considers early- and mid-stages in the development of the bird embryo, up to about Hamburger and Hamilton stage 34. At this point, the shape of the beak is largely set, which coincides with the disappearance of the growth zone at the rostral tip of the beak. The absolute size of the beak appears to change through more uniform cell proliferation into the late stages of embryogenesis and beyond. However, most observations indicate that the shape modulo size is largely unaffected by these processes until adulthood [22] , [23] . The general approach used here to predict shared features of the developmental process over a relatively large phylogenetic range is probably also applicable to other systems or further morphological features in the songbirds. However, the surprisingly simple prediction that growth zone dynamics must be power laws with exponents p / q =2 arises because of two special properties. First, the morphological diversity of the midsagittal plane in the species examined here is low, with only three scalar parameters capturing all shapes. Second, two of these three parameters (length and height) are easily identifiable, and have long been used to quantify basic aspects of beak diversity [15] , [24] , [28] . In general, over deeper phylogenies, we expect beak diversity to require more parameters, weakening the constraints on the developmental process. Studies investigating further aspects of beak diversity (for example, the lower and upper beak [7] , or width in addition to length and height [9] , [10] , [30] ) suggest that the full three-dimensional diversity beyond the midsagittal plane might likewise require a larger number of parameters, perhaps even for the species investigated here. Species where the entire bill curves due to a shifting axis of growth, such as in parrots, cannot yet be fully captured by the model we describe and may require additional developmental mechanisms to explain [18] , [25] . Nonetheless, the general methodology outlined here provides a way to begin to unravel the variability of developmental programmes over a wide phylogeny, even when the number of model organisms through which the developmental process can be explicitly studied is highly limited. In summary, the evolution of biological shapes in general and the adaptive significance of bird beak shapes in particular have been an area of much interest in the literature, with many authors hypothesizing that bird beak shape is heavily optimized for feeding and foraging behaviours [3] , [4] , vocal song structure [26] and other external conditions. The present study significantly limits the potential set of parameters that can be optimized, since the intrinsic developmental pathways place strong constraints on the set of beak shapes that are actually produced. Any optimization can only occur within the subspace of shapes that is readily available to the existing beak developmental pathway. For beaks, the available variability of shapes includes simply changing the linear dimensions (length, depth and width) that have long been used to quantify beak shape diversity [27] , [28] , [29] . Although variability in basic dimensions can have great functional significance, containing, for example, birds that can crack large and hard seeds, such as the large ground finch G. magnirostris , and birds that can forage from flowers, for example, the cactus finch G. scandens , there is no reason to expect a priori that the set of shapes accessible to the developmental programs should include the biomechanics optima. Therefore, our findings are consistent with a hypothesis that beak shapes in the birds we studied thus far are, in fact, biased by the beak morphogenetic process, which is dependent on the controlled growth zone decay despite reported high flexibility in the usage of particular molecular pathways and exact tissue modules in different species of songbirds, including those in our study [11] , [12] , [14] , [20] , [30] , [31] . We argue that beak phenotypic variation in songbirds could be evolving under a strong developmental constraint under its accepted current definitions [6] , [32] , [33] , [34] , [35] . The highly controlled decay of the growth zone strongly suggests the presence of constrained upstream molecular mechanisms. The exact nature of such robust developmental constraints is currently unknown but is probably dependent on the interactions of diffusible morphogens with the competent cells within the growing beak skeletal condensations, for example, cell proliferation-controlled decay in the effective release of the morphogen from the overlying facial ectoderm or feedback loops in the morphogenetic mechanism that gradually shut off the signal and/or signal response [36] , [37] , [38] . Future research should investigate precise molecular controls of the beak growth zone dynamics in multiple bird species with differently shaped beaks to explain the fundamental causes of their beak shape evolution. Sample collection All animal experiments have been approved by the Institutional Biosafety Committee of the Faculty of Arts and Sciences and Committee on Microbiological Safety of Harvard University. Zebra finch eggs were collected from Dr Timothy Gardner’s lab at the Boston University and incubated at 38 °C until they matured to the appropriate stage. Staging of the zebra finch embryos followed the staging system for chicken ( Gallus gallus ) [39] . The staging was broken up into five phases: phase I (embryonic day (E) 5) corresponding to stages 28–29, phase II (E6) to stages 30–31, phase III (E7) to stages 32–33, phase IV (E8) to stages 34–36 and phase V (E9) to stages 37–38. Application of EdU to embryos Before opening a small window on the top of the egg to make access to the embryos possible, 0.1–0.5 ml of albumin (egg white) was removed from the egg with a syringe. To label proliferating cells in the embryos, we used Click-iT EdU Imaging Kit (C10337, Invitrogen). EdU (5-ethynyl-2′-deoxyuridine) is a nucleoside analogue of thymidine and is incorporated into DNA during active DNA synthesis. After perforating the amniotic membrane with sharpened forceps, 20–100 μl of 500 μM EdU in 1 × PBS was dropped over the embryo. The EdU signal was later detected by using a fluorescent azide (Alexa Fluor 488, Invitrogen) to label the EdU with green fluorescence. The eggs were then placed in the incubator at 39 °C for 2–3 h, to allow EdU to be incorporated into the DNA. After taking out the embryos from the eggs, the heads were separated from the bodies and placed in sufficient amount of 4% paraformaldehyde in 1 × PBS solution and stored at 4 °C overnight. The heads were then washed in 1 × PBS for 5 min twice and put through 10% sucrose in 1 × PBS at 4 °C overnight, 30% sucrose in 1 × PBS at 4 °C overnight and 50% optimal cutting temperature (OCT) compound in 30% sucrose/PBS at 4 °C overnight. Then, the heads of embryos were placed in 100% OCT at room temperature for 30 min–2 h. Next, they were embedded in OCT within the cryomolds and flash frozen with dry ice and ethanol, stored at −80 °C until sectioning. Heads were sectioned in the medial plane on a Leica CM 3050S cryostat at −20 °C. The sectioned tissues were placed onto micro slides (VWR, Superfrost Plus) and stored at −80 °C until staining. EdU detection and staining of cartilaginous tissues Once sectioned, EdU detection was performed following the manufacturer’s instruction (Click-iT EdU Imaging Kits, Invitrogen). After detecting EdU in the tissues, cartilaginous tissues were stained following standard protocols. For early stages (phases I and II), Lectin PNA Conjugates (L32459, Molecular Probes) is used to label the cartilage precursors, including that of pnc , in the embryos. For later stages (phases III, IV and V), anti-collagen II polyclonal antibody (ab34712, Abcam) is used to label the differentiated cartilages. Finally, to visualize the cell nuclei, sections were counterstained with a fluorescent blue nuclear stain (Hoechst 33342, Invitrogen). The slides were then washed with PBS and then cover slipped with Fluoromount-G (SouthernBiotech). Measurement of growth zone size For each developmental stage from E5 to E9, we select one section (out of a total of 79) with the clearest and most defined EdU signature near the front of the developing beak. To filter out the EdU signal, we first tone map the RGB channels in Photoshop CS6 (red −70, green +50, blue −20) into a greyscale image, so only cells stained with EdU are visible. To improve contrast, we equalize the histogram in Photoshop CS6 (by manually adjusting levels) to use the full dynamic range at 24 bit depth per pixel. To measure the area of the growth zone, we require a continuous signal; thus, we apply a Gaussian Blur with a radius of ~20 times the average cell centre distance for neighbouring cells (again in Photoshop CS6, see Supplementary Fig. 2 ). The resulting image is then analysed with ImageJ 1.46 by applying a thresholding to the greyscale image (for a range of ~70–255 in brightness, which is manually adjusted to ensure that the signal does not include noise due to points that lie on the epithelium or even outside the beak). Measurement of growth zone speed Comparison between different sections at the same developmental stage indicate that the distance of the growth zone to the commissure (where upper and lower beak meet) is very uniform. In addition, the commissure is just outside the developmental module that will become the upper beak. This distance is thus a good measure for determining the speed with which the growth zone advances. For each growth zone as determined above, we find its centroid, and measure the distance from the commissure to the centroid (both in ImageJ 1.46). Since the increase in distance between different developmental stages is fairly uniform, the growth zone speed can be approximated to high accuracy by v =Δ s /Δ t . Beak shape digitization The shapes used for analysis were from specimens in the Museum of Comparative Zoology at the Harvard University and the American Museum of Natural History in New York. Lateral photographs of museum specimens of each species were taken under slightly underexposed conditions (−1.5 EV) with a Nikon D-90 digital camera. Underexposed photographs allow us to track the silhouette of the bird beak, making the detection of the beak profile more efficient and accurate. Using a feature detection programme (Steerable—ImageJ plugin), we detect the contour of the beak at pixel resolution (pixel size around 10 μm). The beak profile obtained from the feature detection analysis corresponds to a set of points (pixels) in the plane. To obtain a smooth profile of the upper beak, we trace a cubic spline of the upper profile of the beak. This smooth upper beak profile is used for the pairwise comparison of shapes. Beak shape analysis We are interested in quantifying the differences between a given pair of shapes. Specifically, we want to quantify the difference between a reference, unmodified shape y 1 and a beak shape y 2 transformed via a scaling or shear transformation. The obtained outlines (beak shapes) were in Matlab R2011 using the distance metrics E s ( z 1 , z 2 ) and E d ( y 1 , y 2 ) for two real valued functions y 1 and y 2 defined as and where x m is the end point of the beak and corresponds to a scaling transformation with scaling factors s x and s y in the length and depth directions, respectively. The defined measures are dimensionless quantities that depend only on the two scaling factors s x and s y . A necessary condition for two given beak shapes to be related through a scaling transformation is the existence of a minimum of both defined measures, E s and E d , for particular values and of the scaling factors. For the reference and transformed shapes to collapse, landmark points in one shape must also be mapped onto the same landmark points of the other shape. In particular, the beak tip and end point of the beak of the reference shape should coincide with the beak tip and end point in the collapsed shape. This effectively restricts the space of s x and s y that we are allowed to search for a minimum, as previously described [13] , [14] , [20] . Derivation of envelope equation We define the shape of the growth zone by the solution to where and The envelope for these growth zone shapes is given by ∂ t G =0 as where and , for any power laws of the form x 0 ( t )= α ( t *− t ) q , y 0 ( t )= β ( t *− t ) q and l ( t )=γ( t *− t ) p . As a special case, we here consider the growth zone to be elliptical, but the result is more general Then, the equations for the envelope read In this special case, equation (8) implies which can be solved for example, ξ =(1− b Λ η η )/Λ ξ a . This makes equation (9) a quadratic equation in ξ with solutions where Γ 1 and Γ 2 are constants, if α , β , γ , p , q , a , b are chosen. We can express these solutions in terms of the original variables as that can be subtracted to yield and plugging this expression back into equation (8) yields. Monte–Carlo simulations of beak morphogenesis The dynamics outlined in the main text have to be satisfied individually for both the upper and lower profile. However, as shown above, even for a single profile the invariance of beak shapes sets the exponents of the power laws ( p and q ) and the precise shape of the profiles forces values for all other parameters in these power laws ( α , β and γ ). Since the required values for these parameters will generally be slightly different for the upper and lower profile, both can only be satisfied simultaneously if we allow for an additional degree of freedom in allowing the shape of the growth zone (before parameterized by a single parameter l ) to be anisotropic. We expect that only a small set of growth zone shapes can generate a given beak, if the growth zone’s centre is forced to follow a straight line at uniform speed ( q =1) and its dimension perpendicular to the path of motion to shrink in time according to l ∝ t 1/2 , to preserve affine invariance of beak shapes. To find these shapes, we explore beak shapes generated by different growth zone shapes and choices for α , β and γ subject to the dynamics determined before and score the resulting shapes according to their similarity with a given beak profile for one of the species studied here. Monte–Carlo simulations show that indeed only a very small number of growth zone shapes are able to reproduce a prescribed beak shape. For each beak, these effectively fall into a one-parameter family, which is the size of the growth zone when beak development is initiated; see Supplementary Fig. 4 . The generated growth zone shapes agree surprisingly closely with experimentally determined growth zone shapes (compare Fig. 2 with Supplementary Fig. 4 ). We search for growth zone shapes that simultaneously generate a given upper and lower beak profile y u ( x ) and y l ( x )) with a Monte–Carlo simulated annealing approach. It searches for a minimum in the difference between the desired beak shape and the profile ( p u ( x ) and p l ( x )) generated by a fixed growth law and assumed growth zone shape, defined by where φ is a vector parametrizing the shape and all other free parameters in the problem. We quantify an initial growth zone shape by the first k normalized Fourier components b k = a k / a 0 of its centroid distance function is defined by where and for a boundary with N points. The Fourier coefficients are defined as The resulting Fourier components b k are invariant with respect to translation, rotation and scaling, insensitive to noise in the initial data and can encode complex shapes with very few components and are thus ideal to parameterize growth zone shape. To find a minimum, we take random steps d φ in our search space where δ is the rotation angle of the growth zone relative to the x axis, β / α is the slope of the line on which the centroid of the growth zone moves and γ / α parametrizes the scaling of the growth zone size. For this step, we calculate the change in E as Δ E = E ( φ + dφ )− E ( φ ). If Δ E <0, we always accept the step; however, when it is positive, we only accept the step with a probability of p = e −Δ E / T , where T is the annealing temperature. To converge on a minimum, we reduce this temperature T every 15 succesful steps according to a cooling schedule of the form where c is chosen to be substantially larger than any expected Δ E . The size of each random step is chosen dynamically such that we ensure that a significant part of the search space is explored and sufficient information is gained at each temperature (that there is a reasonable ratio of accepted and rejected steps). The search is terminated when a stopping criterion of the form is satisfied, where Ē is the average change in E during the last 15 steps and E min is the minimum during the same number of steps. To ensure that the minimum identified in this manner is indeed a global minimum, we start at three different initial shapes (ellipses with different aspect rations and rotation angles) for each given initial growth zone size and check convergence to the same solution. Phylogeny and ancestral state reconstruction of beak shapes We inferred a phylogeny for Thraupidae using maximum likelihood implemented using RAxML v7.3.1, accessed via the CIPRES Science Gateway v3.1 (refs 40 , 41 , 42 ). Our data set included 359 species that were sampled for up to six genes per species including two mitochondrial genes ( cyt b and ND2 ), two nuclear introns (FGB-I5 and MB-I2), a protein-coding nuclear gene ( RAG1 ) and a sex-linked nuclear gene ( AC01-I9 ). The data set was partitioned by gene and codon position when applicable for coding regions, resulting in 12 partitions; RAxML applies a GTR+G model to each partition. We pruned the most likely tree [43] to include only those species for which we had reliable beak data from multiple museum specimens ( Fig. 1 ). The other phylogenies shown in Fig. 1 are based on previously published results for Passeroidea [44] , Cardinalidae [45] , [46] , [47] and Estrildidae [48] , [49] . Beak shapes were mapped onto the phylogeny using maximum likelihood with Mesquite v2.75. Illustrations of bird head shown in Fig. 1 were reproduced from ref. 50 with permission. How to cite this article: Fritz, J. A. et al . Shared developmental programme strongly constrains beak shape diversity in songbirds. Nat. Commun. 5:3700 doi: 10.1038/ncomms4700 (2014).